Direct measurement of discrete valley and orbital quantum numbers in bilayer graphene The high magnetic field electronic structure of bilayer graphene is enhanced by the spin, valley isospin, and an accidental orbital degeneracy, leading to a complex phase diagram of broken symmetry states. Here, we present a technique for measuring the layer-resolved charge density, from which we directly determine the valley and orbital polarization within the zero energy Landau level. Layer polarization evolves in discrete steps across 32 electric field-tuned phase transitions between states of different valley, spin, and orbital order, including previously unobserved orbitally polarized states stabilized by skew interlayer hopping. We fit our data to a model that captures both single-particle and interaction-induced anisotropies, providing a complete picture of this correlated electron system. The resulting roadmap to symmetry breaking paves the way for deterministic engineering of fractional quantum Hall states, while our layer-resolved technique is readily extendable to other two-dimensional materials where layer polarization maps to the valley or spin quantum numbers. The single-particle energy spectrum of a two-dimensional electron system (2DES) in a large magnetic field collapses into Landau levels (LLs) containing N Φ degenerate states, with N Φ the number of magnetic flux quanta penetrating the sample. The width in energy of the LL bands is limited only by disorder, making electronic interactions effectively strong in a clean system even when their absolute scale is weak. The simplicity of the starting LL wavefunctions, combined with the high degree of control available in 2DES, make LLs a promising venue for engineering electronic ground states based on electron correlations. However, the difficulty of simulating interacting electron problems necessitates experimental input to constrain the possible ground states, particularly in the presence of internal degeneracy. The Bernal bilayer graphene (B-BLG) zero energy Landau level (ZLL) provides an extreme example of such degeneracy. In B-BLG, LLs \(\left| {\xi N\sigma } \right\rangle \) are labeled by their electron spin σ = ↑, ↓, valley ξ = +, −, and orbital index \(N \in {\Bbb Z}\) . Electrons in valley +/− are localized near points K / K ′ of the hexagonal Brillouin zone, while the index N is closely analogous to the LL-index of conventional LL systems. The energies of the LLs are approximately \({\epsilon _{\sigma \xi N}} \approx \hbar {\omega _c}{\rm{sign}}\left( N \right)\sqrt {N\left( {N - 1} \right)} \) , where ħω c is the cyclotron energy, leading to an eight-fold nearly degenerate ZLL comprising the N = 0 and N = 1 orbitals and all possible spin and valley isospin combinations. While direct probes of spin in 2DESs were demonstrated two decades ago [1] , the valley quantum number has only been probed indirectly in semiconductor quantum wells [2] , graphene monolayer [3] , [4] and bilayers [5] , [6] , [7] , [8] , [9] , [10] , [11] , [12] , [13] , and transition metal dichalcogenides [14] . In bilayer graphene, resolving the order in which the eight components fill as electrons are added is one of the key open questions, and is essential to efforts to use bilayer graphene to engineer exotic phases of matter based on electronic correlations [15] , [16] . Due to an approximate SU(4) symmetry relating spin and valley, determining which of the components are filled is non-trivial. Past experiments [5] , [6] , [7] , [8] , [9] , [10] , [11] , [12] , [13] , [17] have observed numerous phase transitions between gapped ground states at both integer [6] , [7] , [8] , [9] , [12] , [13] , [17] and fractional [10] , [11] , [13] filling. However, these experiments are insufficient to constrain realistic theoretical models, in which the preferred ordering is determined by a combination of the Zeeman energy, which splits the spins; Coulomb interactions and band structure effects, both of which distinguish between the N = 0, 1 orbitals; and several small valley anisotropies which weakly break the valley-SU(2) symmetry [18] , [19] , [20] , [21] , [22] , [23] , [24] . Indeed, two recent experimental papers explain their data using mutually contradictory single-particle [12] and purely interacting pictures [10] . Constructing a more complete theory of symmetry breaking in bilayer graphene requires experimental determination of the partial filling of each spin, valley, and orbital level, \({\nu _{\xi N\sigma }} = \langle {\hat N_{\xi N\sigma }^e} \rangle {\rm{/}}{N^\Phi }\) as it evolves with total LL filling. In this work, we introduce a direct measurement of two out of three of these components, by exploiting the fact that the four valley and orbital components indexed by ξN have different weights on the two layers of the bilayer. We detect this difference in layer polarization capacitively, and use it to infer the fillings ν ξN as a function of both the total electron density and applied perpendicular electric field. Layer polarization measurements Our devices consist of hexagonal boron nitride encapsulated B-BLG flakes [25] fitted with metal top and bottom gates (Fig. 1a, b ). The layer polarization and total charge density are tuned by a combination of applied top and bottom gate voltages ( v t and v b ), expressed through their symmetric and antisymmetric combinations n 0 ( p 0 ) ≡ c t v t ± c b v b with c t(b) the geometric capacitances between the respective gates and the B-BLG. − n 0 and − p 0 correspond to the induced charge density and layer polarization in the limit of a perfectly metallic, infinitesimally spaced bilayer. Generically, the physically realized total density ( n ) and layer density imbalance ( p ) deviate from this limit, particularly at high magnetic fields. A simple electrostatic model (Supplementary Note 1 ) shows that these deviations manifest as corrections to the measured gate capacitances ( C T and C B ) as 
    C_S≡C_T + C_B = 2c∂ n/∂n_0
 (1) 
    C_A≡C_T - C_B = 2c∂ n/∂p_0 = c^2/c_0∂ p/∂n_0,
 (2) where c = ( c t + c b )/2 ≈ 1.36 fF/μm 2 and c 0 is the interlayer capacitance of the bilayer. The antisymmetric combination C A is unique to bilayer systems, vanishing identically in a monolayer system, allowing us to measure the layer polarization p . Measuring C A is technically challenging, as it arises from series combination of the large interlayer capacitance and the comparatively small gate capacitance. It is imperative that the dielectric layers be highly uniform across the device, that the areal mismatch between top and bottom gate be kept \( \ll 1\% \) , and the geometric capacitance of the two gates be nearly the same; these requirements are difficult to satisfy in conventional two-dimensional electron bilayers but are readily achieved using single-crystal hBN gate dielectrics and atomically thin bilayers. Fig. 1 Layer polarization of bilayer graphene at zero magnetic field. a Measurement schematic showing geometric gate capacitances c t and c b and interlayer capacitance c 0 . Capacitance is measured using a cryogenic bridge circuit by comparison with a standard capacitor C std , measured to be 404 ± 20 fF (see “Methods”). b Device image. Top gate (TG), back gate (BG), and contacts to bilayer graphene (G) are shown. Scale bar is 10 μm; device area is approximately 87 μm 2 . c C S measured at B = 0 and T = 1.6 K as a function of n 0 / c = v t + v b and p 0 / c = v t − v b . A p 0 -dependent band gap is visible as the dark region near n 0 = 0. d Line traces taken at different values of p 0 , corresponding to dashed lines in c . Band edge van Hove singularities [28] and electron-hole asymmetry [27] are both evident. e C A measured under the same conditions. A common, constant background has been subtracted to account for fixed parasitic capacitances. f Line traces at different values of p 0 corresponding to dashed lines in e . g Integrated change in polarization, \(\frac{{{c_0}}}{c}{\int} {{C_A}{\kern 1pt} d\left( {\frac{{{n_0}}}{c}} \right) = \Delta p} \) , with the constant of integration fixed to be zero at high \(\left| {{n_0}} \right|\) . 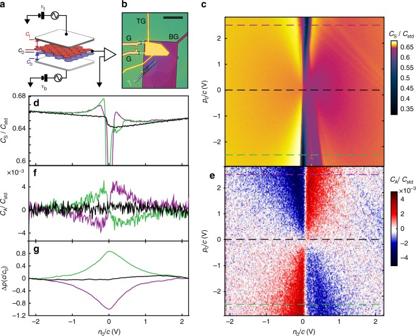Fig. 1 Layer polarization of bilayer graphene at zero magnetic field.aMeasurement schematic showing geometric gate capacitancesctandcband interlayer capacitancec0. Capacitance is measured using a cryogenic bridge circuit by comparison with a standard capacitorCstd, measured to be 404 ± 20 fF (see “Methods”).bDevice image. Top gate (TG), back gate (BG), and contacts to bilayer graphene (G) are shown.Scale baris 10 μm; device area is approximately 87 μm2.cCSmeasured atB= 0 andT= 1.6 K as a function ofn0/c=vt+vbandp0/c=vt−vb. Ap0-dependent band gap is visible as the dark region nearn0= 0.dLine traces taken at different values ofp0, corresponding todashed linesinc. Band edge van Hove singularities28and electron-hole asymmetry27are both evident.eCAmeasured under the same conditions. A common, constant background has been subtracted to account for fixed parasitic capacitances.fLine traces at different values ofp0corresponding todashed linesine.gIntegrated change in polarization,\(\frac{{{c_0}}}{c}{\int} {{C_A}{\kern 1pt} d\left( {\frac{{{n_0}}}{c}} \right) = \Delta p} \), with the constant of integration fixed to be zero at high\(\left| {{n_0}} \right|\). In accordance with single-particle band structure28, wavefunctions are layer unpolarized forp0= 0, while for large\(\left| {{p_0}} \right|\)the polarization peaks atn0= 0, where band wavefunctions are strongly layer polarized In accordance with single-particle band structure [28] , wavefunctions are layer unpolarized for p 0 = 0, while for large \(\left| {{p_0}} \right|\) the polarization peaks at n 0 = 0, where band wavefunctions are strongly layer polarized Full size image Figure 1c and e show C S and C A measured at zero magnetic field as a function of n 0 and p 0 . The C S data are dominated by quantum capacitance features of the B-BLG band structure, which features a quadratic band touching at low energies and hyperbolic bands at high energies [26] . An electric field ( p 0 ) opens a band gap with \(\sqrt \epsilon \) van Hove singularities at the band edges, as can be readily seen in the experimental data (Fig. 1d ). Although C S is approximately particle-hole symmetric, significant symmetry breaking contributions are evident. We attribute this to the skew interlayer hopping parameter γ 4 in the Slonczewski-Weiss-McClure model for graphite, which breaks particle-hole symmetry by making the lattice non-bipartite (Supplementary Fig. 4 ) [27] . C A data, in contrast, reflect the layer-resolved properties of the band wavefunctions (Fig. 1e, f ). For p 0 ≠ 0, wavefunctions are layer-polarized near the band extrema, so that the first electrons or holes added to the neutral system are added to the corresponding low-energy layer. Reversing p 0 inverts the role of the top and bottom layers, inverting the sign of the measured signal with respect to n 0 . At high overall electron density, the applied p 0 is fully screened, so that charge is added symmetrically to the two layers [28] . The relative layer polarization at different values of n 0 can then be extracted by integrating Eq. ( 2 ) with respect to n 0 (Fig. 1g ). 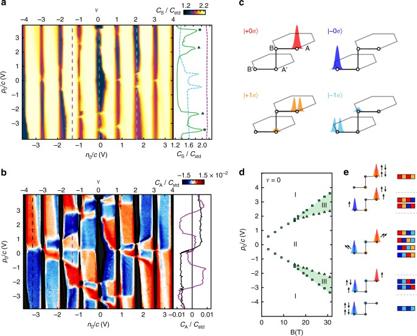Fig. 2 Valley and orbital polarization of the ZLL.aLayer-symmetric capacitance\({C_{\rm{S}}} \propto \frac{{\partial n}}{{\partial {n_0}}}\)atT= 300 mK andB= 31 T. Incompressible states manifest as drops inCS(black) at all integer fillingsν. Phase transitions between different valley and orbital fillings at fixedνmanifest as compressible spikes, as shown in the side panel forν= 0 (green,solid) andν= 2 (light blue,dashed). A total of 16 phase transitions are observed at integerν, with one each atν= ±3, two atν= ±2, three atν= ±1, and four atν= 0. No experimental contrast is visible at non-integer filling (purple,dashed).bLayer-antisymmetric capacitance\({C_{\rm{A}}} \propto \frac{{\partial p}}{{\partial {n_0}}}\)atT= 300 mK andB= 31 T.Blackregions mask portions of the parameter space with large dissipation inCS, which arises when a large gap leads to a low in-plane conductivity and failure to charge regions of the sample during a ~13 μs measurement cycle (see “Methods”). The color scheme highlights the 4-tone contrast, interpreted as filling of\(\left| {\xi N\sigma } \right\rangle \)=\(\left| { + 0\sigma } \right\rangle \)(red),\(\left| { + 1\sigma } \right\rangle \)(orange),\(\left| { - 0\sigma } \right\rangle \)(blue), and\(\left| { - 1\sigma } \right\rangle \)(cyan) LLs.cSchematic depiction of the four single-particle wavefunctions |ξNσ〉, showing their relative support on the four atomic sitesA,B,A′, andB′ of the bilayer graphene unit cell. While the\(\left| { + 0\sigma } \right\rangle \)levels are fully polarized (α0= 1), we calculateα1= 0.63 for the\(\left| { + 1\sigma } \right\rangle \).dPhase diagram of gapped states atν= 0. Points are experimentally determined by measuring peaks inCS, as ina(green dashed line), for 0 <B< 31 T. At highB≳15 T an intermediate phase III emerges between the layer-unpolarized canted antiferromagnetic phase II and the layer-polarized phase I6,8.eSchematics of the layer, orbital, and spin polarizations of phases I, II, and III and the ten distinct filling sequences that determine the three valley and orbital polarizations of phases I, II, and III. These sequences are extracted from Fig.2b, filling fromν= −4 toν= 0 over the full range −4V<p0/c< 4V Layer polarization at high magnetic field Figure 2a shows C S measured in the same device at B = 31 T in the ZLL. We observe insulating states at all integer LL filling factors ν , which are characterized by low capacitance C S and high dissipation (see Supplementary Figs. 1 , 2 for dissipation data). Adjusting p 0 / c at fixed integer ν drives transitions characterized by a spike in C S indicating increased conductivity [11] and compressibility, consistent with a closing of the charge gap. Sixteen such phase transitions are evident in the C S data. Similar transitions have been reported in the literature: ref. [6] reported phase transitions at ν = ±2 and p 0 = 0, as well as a single phase transition at ν = 0 and finite p 0 . More recently, the p 0 = 0 transitions at ν = ±1, ±3 are evident in ref. [11] , while the splitting of the p 0 = 0 phase transition at ν = ±2 suggests the formation of a stable, gapped, layer unpolarized state in the region p 0 ~0, as was reported in refs. [9] , [11] . Only in ref. [12] was a potential gapped phase observed at intermediate p 0 and ν = 0. However, a unified framework for understanding the diverse competing phases has not yet emerged. Fig. 2 Valley and orbital polarization of the ZLL. a Layer-symmetric capacitance \({C_{\rm{S}}} \propto \frac{{\partial n}}{{\partial {n_0}}}\) at T = 300 mK and B = 31 T. Incompressible states manifest as drops in C S ( black ) at all integer fillings ν . Phase transitions between different valley and orbital fillings at fixed ν manifest as compressible spikes, as shown in the side panel for ν = 0 ( green , solid ) and ν = 2 ( light blue , dashed ). A total of 16 phase transitions are observed at integer ν , with one each at ν = ±3, two at ν = ±2, three at ν = ±1, and four at ν = 0. No experimental contrast is visible at non-integer filling ( purple , dashed ). b Layer-antisymmetric capacitance \({C_{\rm{A}}} \propto \frac{{\partial p}}{{\partial {n_0}}}\) at T = 300 mK and B = 31 T. Black regions mask portions of the parameter space with large dissipation in C S , which arises when a large gap leads to a low in-plane conductivity and failure to charge regions of the sample during a ~13 μs measurement cycle (see “Methods”). The color scheme highlights the 4-tone contrast, interpreted as filling of \(\left| {\xi N\sigma } \right\rangle \) = \(\left| { + 0\sigma } \right\rangle \) ( red ), \(\left| { + 1\sigma } \right\rangle \) ( orange ), \(\left| { - 0\sigma } \right\rangle \) ( blue ), and \(\left| { - 1\sigma } \right\rangle \) ( cyan ) LLs. c Schematic depiction of the four single-particle wavefunctions | ξNσ 〉, showing their relative support on the four atomic sites A , B , A ′, and B ′ of the bilayer graphene unit cell. While the \(\left| { + 0\sigma } \right\rangle \) levels are fully polarized ( α 0 = 1), we calculate α 1 = 0.63 for the \(\left| { + 1\sigma } \right\rangle \) . d Phase diagram of gapped states at ν = 0. Points are experimentally determined by measuring peaks in C S , as in a ( green dashed line ), for 0 < B < 31 T. At high B ≳ 15 T an intermediate phase III emerges between the layer-unpolarized canted antiferromagnetic phase II and the layer-polarized phase I [6] , [8] . e Schematics of the layer, orbital, and spin polarizations of phases I, II, and III and the ten distinct filling sequences that determine the three valley and orbital polarizations of phases I, II, and III. These sequences are extracted from Fig. 2b , filling from ν = −4 to ν = 0 over the full range −4 V < p 0 / c < 4 V Full size image In contrast to layer-insensitive capacitance [5] , [10] , [12] and transport [6] , [7] , [8] , [9] , [11] measurements, C A provides high experimental contrast throughout the n 0 − p 0 plane (Fig. 2b ). Strikingly, the measured C A falls into discrete levels, corresponding to blue , cyan , orange , and red on the color scale of Fig. 2b . The transitions observed in C S at integer filling fall on lines in the n 0 − p 0 plane along which the sign of C A changes abruptly. To understand the color scale quantitatively, we compute the layer polarization of the ZLL single-particle eigenstates. B-BLG has a 4-site unit cell, with sites A , B in the top layer and A ′, B ′ in the bottom (see Fig. 2c ), and hence the ZLL wavefunctions decompose into their components on the four sublattices, Ψ ( x ) = ( ϕ A ( x ), ϕ B ′ ( x ), ϕ B ( x ), ϕ A ′ ( x )). The layer polarization \({\alpha _{\xi N\sigma }} \equiv {\int} {{d^2}x\left| {{\phi _A}{{(x)}^2}} \right| + \left| {{\phi _B}{{(x)}^2}} \right| - \left| {{\phi _{A'}}{{(x)}^2}} \right| - \left| {{\phi _{B'}}{{(x)}^2}} \right|} \) is constant across all states in a LL, and independent of spin. It has opposite sign in the two valleys [26] , so that positive and negative C A correspond to filling valley K and K ′, and its magnitude depends on the orbital quantum number, so that α ξNσ = ξα N . At B = 31 T, band structure calculations [29] show that α 0 = 1 and α 1 = 0.63. As electrons enter LL \(\left| {\xi N\sigma } \right\rangle \) they contribute a polarization whose magnitude and sign depend on the level being filled. Since \({C_A} \propto \frac{{\partial p}}{{\partial {n_0}}}\) , where n 0 is very nearly the electron density, we thus interpret red, orange, blue, and cyan as indicating regions where electrons are filling \(\left| {\xi N} \right\rangle \) = \(\left| { + 0} \right\rangle \) , \(\left| { + 1} \right\rangle \) , \(\left| { - 0} \right\rangle \) , and \(\left| { - 1} \right\rangle \) type LLs, respectively. This supports a scenario in which, away from phase boundaries, only one of these LLs is filling at each particular ( n 0 , p 0 ). Indeed, numerical calculations (see Supplementary Fig. 5 ) show that as isospin ξσ fills, around 90% of the electrons enter into either the N = 0 or N = 1 orbital; e.g., either \(\frac{{\partial {\nu _{\xi 0\sigma }}}}{{\partial \nu }}{\kern 1pt} \) ≳ 0.9 or \(\frac{{\partial {\nu _{\xi 1\sigma }}}}{{\partial \nu }}{\kern 1pt} \) ≳ 0.9, according to whether the region is red/blue or orange/cyan, respectively. The polarization of all gapped integer states can now be obtained by summing the level filling sequence starting from the ν = −4 vacuum. Consider ν = 0, where five incompressible states are visible in C S (Fig. 2d ). The order in phase I, at large p 0 > 0, can be inferred from the observed C A sequence of red, orange, red, orange, implying two N = 0 and two N = 1 states are filled in valley ξ = +. Its layer-inverse occurs in valley ξ = − for large p 0 < 0. The phase I states are fully valley polarized, and hence spin and orbitally unpolarized due to Pauli exclusion. Phase II, at p 0 near zero, fills levels \(\left| { + 0} \right\rangle ,\left| { + 1} \right\rangle ,\left| { - 0} \right\rangle ,\left| { - 1} \right\rangle \) . A state which fills both orbitals of opposite valleys is consistent with the canted anti-ferromagnetic state [8] , [22] ; however, from C A alone we cannot infer whether the spins are polarized or canted. Finally, phase III at intermediate \(\left| {{p_0}} \right|\) fills levels ±0, ±1, ±0, ∓ 0. The orbital and valley filling sequences derived from Fig. 2b provide a more stringent set of constraints on theoretical models than the integer phase transitions alone. For example, a single particle, four-band tight-binding model accounts for the correct number of integer ν transitions [12] but fails when compared to the C A filling sequence. The single-particle energies of the ZLL, 
    E_ξ Nσ^(1) = - E_Zσ + NΔ _10 - u/2ξα _N
 (3) are shown in Fig. 3a for B = 31 T. Here, E Z is the Zeeman energy, u is the potential across the bilayer, and Δ 10 ∝ γ 4 B is the splitting between the N = 0, 1 orbitals, which arises because particle-hole symmetry no longer pins the ZLL energies to zero. The interlayer bias u ∝ p 0 couples to the differing layer polarization of each state, ξα N , leading to u -tuned crossings at integer fillings; however, the single-particle picture predicts that N = 0 levels fill first for all but the very highest u (Fig. 3b, e ), and the transitions would have zero slope in the n 0 − p 0 plane. This disagrees with the experimental C A data where N = 0 and N = 1 states of the same valley often fill in sequence, and several transition lines have a significant slope. Fig. 3 Theoretical model of spin, valley, and orbital anisotropies in the ZLL. a Single-particle energy spectrum of the ZLL at B = 31 T derived from a four-band tight binding model [29] (see also Eq. ( 3 )). The interlayer potential u couples to the layer polarization of each state as ξα N u , differing in sign for the two valleys and magnitude for the two orbitals; the spin degeneracy is lifted by the Zeeman energy E Z ≈ 3.6 meV; and the N = 0 and 1 orbitals are split by the band structure parameter Δ 10 ≈ 9.7 meV. b – d Level filling schematic for \(\frac{{{p_0}}}{c} = - 100\) mV. Within the Hartree-Fock approximation, we calculate the energy to add an additional electron to level σξN given the current filling { ν σξN }, generating eight curves ε σξN ( ν ) which change with the total filling ν . Colors indicate the ξN index of the level, while solid vs. dashed indicates the spin. The bold portion indicates the range of ν over which the level is coincident with the Fermi energy. As isospin σξ fills, both of its N = 0 and 1 orbitals decrease in energy due to favorable Coulomb correlations, while the components of the opposite valley (i.e., layer) decrease slightly in energy due to the capacitance of the bilayer. The relative magnitude of these effects, combined with the single-particle splittings, determines the filling order, shown here for three interactions strengths parameterized by the boron nitride dielectric constant, \(\epsilon _{{\rm{BN}}}^{||}\) . Large \(\epsilon _{{\rm{BN}}}^{{\rm{||}}} = 18\) ( e ) corresponds to negligible Coulomb interactions, \(\epsilon _{{\rm{BN}}}^{{\rm{||}}} = 6.6\) ( f ) corresponds to intermediate Coulomb interactions, and \(\epsilon _{{\rm{BN}}}^{||} = 1\) ( g ) corresponds to maximally strong Coulomb interactoins. e – g Hartree-Fock phase diagram in the three interaction strength regimes. 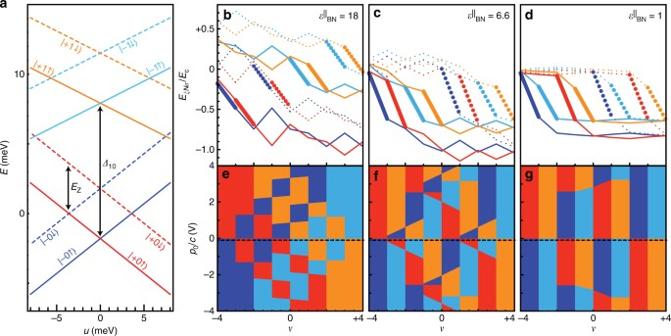Fig. 3 Theoretical model of spin, valley, and orbital anisotropies in the ZLL.aSingle-particle energy spectrum of the ZLL atB= 31 T derived from a four-band tight binding model29(see also Eq. (3)). The interlayer potentialucouples to the layer polarization of each state asξαNu, differing in sign for the two valleys and magnitude for the two orbitals; the spin degeneracy is lifted by the Zeeman energyEZ≈ 3.6 meV; and theN= 0 and 1 orbitals are split by the band structure parameter Δ10≈ 9.7 meV.b–dLevel filling schematic for\(\frac{{{p_0}}}{c} = - 100\)mV. Within the Hartree-Fock approximation, we calculate the energy to add an additional electron to levelσξNgiven the current filling {νσξN}, generating eight curvesεσξN(ν) which change with the total fillingν.Colorsindicate theξNindex of the level, whilesolidvs.dashedindicates the spin. Thebold portionindicates the range ofνover which the level is coincident with the Fermi energy. As isospinσξfills, both of itsN= 0 and 1 orbitals decrease in energy due to favorable Coulomb correlations, while the components of the opposite valley (i.e., layer) decrease slightly in energy due to the capacitance of the bilayer. The relative magnitude of these effects, combined with the single-particle splittings, determines the filling order, shown here for three interactions strengths parameterized by the boron nitride dielectric constant,\(\epsilon _{{\rm{BN}}}^{||}\). Large\(\epsilon _{{\rm{BN}}}^{{\rm{||}}} = 18\)(e) corresponds to negligible Coulomb interactions,\(\epsilon _{{\rm{BN}}}^{{\rm{||}}} = 6.6\)(f) corresponds to intermediate Coulomb interactions, and\(\epsilon _{{\rm{BN}}}^{||} = 1\)(g) corresponds to maximally strong Coulomb interactoins.e–gHartree-Fock phase diagram in the three interaction strength regimes. Colorsblue,cyan,red, andorangeindicate whether levels of typeξN= −0, −1, +0, +1 are filling, so that the result should mimic the observedCA. The intermediate interaction regime shows good agreement with the experimentalCAdata, while interactions which are too weak (e) or strong (g) do not reproduce the observed filling sequences. Theblack dashed lineindicates a cut atp0/c= −100 meV corresponding to the particular filling sequence shown inb–d Colors blue , cyan , red , and orange indicate whether levels of type ξN = −0, −1, +0, +1 are filling, so that the result should mimic the observed C A . The intermediate interaction regime shows good agreement with the experimental C A data, while interactions which are too weak ( e ) or strong ( g ) do not reproduce the observed filling sequences. The black dashed line indicates a cut at p 0 / c = −100 meV corresponding to the particular filling sequence shown in b – d Full size image The departure from the single-particle picture arises from the failure to account for the Coulomb interaction, which both favors sequential filling of N = 0, 1 levels of the same isospin due to exchange [18] , [19] and penalizes valley polarization due to the interlayer capacitance of the bilayer. However, if Coulomb correlations are made too strong, the first effect dominates and N = 0, 1 orbitals of an isospin always fill sequentially, as shown in Fig. 3d and g . Apparently, competition between the splitting Δ 10 and Coulomb correlations is essential. To determine whether a single model can account for all the observed phase boundaries, we analyze a model that accounts for the single-particle splittings, the SU(4)-invariant screened Coulomb interaction, and several subleading valley anisotropies (Supplementary Note 2 ). Evaluating the model within a Hartree-Fock approximation allows us to compute the energies of the competing filling sequences, and thereby determine their phase boundaries in the n 0 − p 0 plane. The model depends on three phenomenological constants (a screening strength, the perpendicular dielectric constant of the BLG, and a valley anisotropy), which we can now estimate by matching the location of the integer transitions and their dependence on an in-plane B -field. The resulting phase diagram is shown in Fig. 3c , and shows good agreement with the C A data of Fig. 2b , including the location of the transitions in absolute units of p 0 / c and several of their slopes. In our model, each integer state is obtained by fulfilling some number of ξNσ levels; in particular it does not require interlayer coherent phases that spontaneously break the valley U(1) × U(1) symmetry, in contrast to theories that predict such phases at ν = ±1, p 0 = 0. We also predict that the ν = 0 phase III observed at ν = 0 likely hosts helical edge states similar to those recently described in twisted bilayer graphene [30] . This state is stabilized by the single-particle anisotropy Δ 10 and antagonized by the Coulomb interactions, suggesting it could be further stabilized in devices with stronger screening due to proximal metal gates. Despite good overall agreement, there is an interesting qualitative discrepancy between the Hartree-Fock analysis and the data. In the experiment, the slope of the phase transition line between −2 < ν < −1 (see Fig. 4a , boundary (ii)–(iv)) is significantly larger than the slope of the adjoining transition across −3 < ν < −2 (boundary (i)–(iii) of Fig. 4a ). Within the Hartree-Fock approximation, the slopes are identical, and in fact any model which neglects scattering (e.g., “Landau-level mixing”) between the N = 0, 1 orbitals has a particle-hole symmetry ν + 2 → −( ν + 2), u − u * ( ν = −2) → −( u − u * (−2)), forcing the two boundaries to mirror each other. 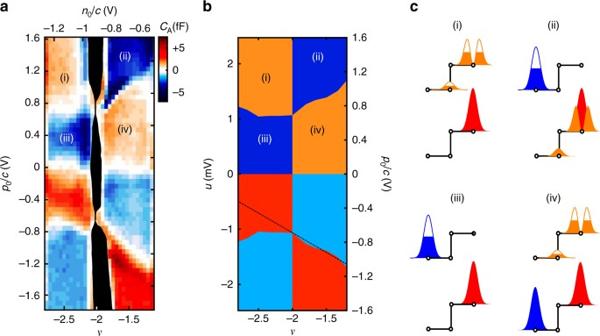Fig. 4 Correlation effects at partial LL filling.aDetail ofCAnearν= −2. Sign changes inCAas a function ofn0indicate polarization extrema and phase transitions. The strong dependence of the phase transition lines onνare a consequence of interactions, which cause the energy per particle of the competing phases to depend onν.bPhase diagram from multicomponent infinite DMRG calculations31for a four-band model of bilayer graphene with Coulomb interactions. In contrast to the Hartree-Fock prediction shown in Fig.3c, experiments show that the magnitude of the slope of the phase boundary between (i) and (iii) differs from the boundary betweem (ii) and (iv). This implies that strong scattering between theN= 0, 1 orbitals breaks the particle-hole symmetryν↔ −(ν+ 2), an effect which is correctly accounted for in our DMRG simulations.cSchematic representation of the four phases appearing ina. Each of the four orbital typesξNdepicted in Fig.2ccan either be filled (solid, shown inbottom unit cell), or in the process of filling (partially solid, shown intop unit cell). Phase (ii), for example, consists of fully filled\(\left| { + 0} \right\rangle \)and\(\left| { + 1} \right\rangle \)levels, while level\(\left| { - 0} \right\rangle \)is filling 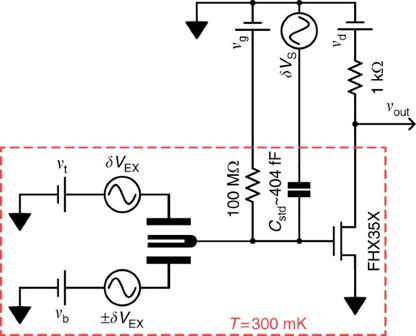Fig. 5 Electrical schematic of the capacitance measurement. DC voltagesvt,vbandvgtogether controln0andp0, with fixedvg≈ −300 mV such that the transistor amplifier is at its optimal working point. ForCSmeasurements, an AC excitationδVEXis applied to both top and bottom gate.δVSis then chosen to balance the bridge for a single set of DC voltages, i.e., such thatδvout= 0, in which caseCS/Cstd=δVS/δVEX.n0andp0are then swept andδvoutmonitored, from whichCS(n0,p0) is extracted. ForCA, the measurement proceeds identically but with opposite phase signals applied to the two gates To account for the asymmetry, we instead find the ground state of the model’s Hamiltonian using the multicomponent infinite-density matrix renormalization group, which takes full account of correlations [31] . Allowing LL mixing produces a kink in the slope at ν = −2, as experimentally observed (Fig. 4b ). LL mixing is known to generate effective three-body interactions, which stabilize fractional non-Abelian phases [32] , [33] ; our results suggest that these interactions may be stronger in BLG than in conventional semiconductor quantum wells. Fig. 4 Correlation effects at partial LL filling. a Detail of C A near ν = −2. Sign changes in C A as a function of n 0 indicate polarization extrema and phase transitions. The strong dependence of the phase transition lines on ν are a consequence of interactions, which cause the energy per particle of the competing phases to depend on ν . b Phase diagram from multicomponent infinite DMRG calculations [31] for a four-band model of bilayer graphene with Coulomb interactions. In contrast to the Hartree-Fock prediction shown in Fig. 3c , experiments show that the magnitude of the slope of the phase boundary between (i) and (iii) differs from the boundary betweem (ii) and (iv). This implies that strong scattering between the N = 0, 1 orbitals breaks the particle-hole symmetry ν ↔ −( ν + 2), an effect which is correctly accounted for in our DMRG simulations. c Schematic representation of the four phases appearing in a . Each of the four orbital types ξN depicted in Fig. 2c can either be filled ( solid , shown in bottom unit cell ), or in the process of filling ( partially solid , shown in top unit cell ). Phase (ii), for example, consists of fully filled \(\left| { + 0} \right\rangle \) and \(\left| { + 1} \right\rangle \) levels, while level \(\left| { - 0} \right\rangle \) is filling Full size image In conclusion, we have described a new experimental technique to determine the layer polarization of van der Waals bilayers and used it to constrain a detailed model of symmetry breaking in the bilayer graphene ZLL. Our technique is readily applicable to quantitatively probe layer, valley, and spin polarization in other atomic layered materials, including twisted bilayer graphene and both homobilayer and heterobilayer of transition metal dichalcogenides. Sample preparation Bilayer graphene samples encapsulated in hexagonal boron nitride were fabricated using a dry transfer method [25] . Particular care is taken to ensure that the top and bottom hBN flakes are of the same thickness, measured by atomic force microscopy to be 19 and 20 nm, respectively. During fabrication, care is also taken to minimize the area of graphene bilayer gated by only one of the two gates, as single-gated areas contribute a systematic error to the measured C A signal proportional to the area and to C S . Anticipating \(\frac{{{C_A}}}{{{C_S}}} \approx \frac{c}{{2{c_0}}}\) ≲ \(\frac{{3.35\,{\rm{A}}}}{{39\,{\rm{nm}}}} = .0086\) , we ensure that the areal mismatch between bottom-gated and top-gated areas is less than .5%. Capacitance measurement electrical schematic Capacitance measurements were made using a cryogenic impedance transformer based on an FHX35X high electron mobility transistor [34] in a bridge configuration connected to the bilayer graphene ohmic contacts (see Fig. 5 ). v g sets the transistor bias point and v d adjusted to be sufficiently low that no sample heating is observed. To measure C S(A) , two synchronized and nearly equal-magnitude AC signals ( δV EX ) are applied to the top and bottom gates, whose relative magnitude is chosen to match the ratio of geometric capacitances c t / c b extracted from the DC characteristics of the device. The signals are applied in phase for C S and out of phase for C A . A third AC signal is applied to a standard capacitor C std with amplitude and phase that null the signal at the input of the cryogenic amplifier, and the capacitance and dissipation determined from the relation of the AC signals. C std was measured to be 404 fF during the cooldown in which the data of Fig. 1 were measured. We used this value to determine C S and C A shown in subsequent figures, although in our experience C std can vary by up to 20 fF from cooldown to cooldown, thus introducing a systematic uncertainty of approximately 5% in the capacitance shown in Figs. 2 – 4 . All data shown are acquired off-balance, by monitoring the voltage at the balance point as DC values of the gate voltages are changed. Data in Fig. 2a and b are measured at 67.778 kHz using a 10 mV variation of n 0 / c and of p 0 / c , respectively. Fig. 5 Electrical schematic of the capacitance measurement. DC voltages v t , v b and v g together control n 0 and p 0 , with fixed v g ≈ −300 mV such that the transistor amplifier is at its optimal working point. For C S measurements, an AC excitation δV EX is applied to both top and bottom gate. δV S is then chosen to balance the bridge for a single set of DC voltages, i.e., such that δv out = 0, in which case C S / C std = δV S / δV EX . n 0 and p 0 are then swept and δv out monitored, from which C S ( n 0 , p 0 ) is extracted. For C A , the measurement proceeds identically but with opposite phase signals applied to the two gates Full size image Interpretation of C A as a thermodynamic derivative requires that the sample is sufficiently conductive to fully charge over a time scale comparable to the inverse measurement frequency [35] . At low temperature and high magnetic fields, our sample becomes strongly insulating at integer filling factors, precluding this condition being satisfied. Failure to charge manifests as an increase in the out of phase, dissipative signal in the capacitance, allowing us to monitor charging across the parameter range. In Figs. 2 b and 4a , regions in which the sample does not charge are masked in black , and dissipation data for all data sets is shown in Supplementary Figs. 1 and 2 . Data availability The data that support the findings of this study are available from the corresponding author upon reasonable request.